Effectors of animal and plant pathogens use a common domain to bind host phosphoinositides Bacterial Type III Secretion Systems deliver effectors into host cells to manipulate cellular processes to the advantage of the pathogen. Many host targets of these effectors are found on membranes. Therefore, to identify their targets, effectors often use specialized membrane-localization domains to localize to appropriate host membranes. However, the molecular mechanisms used by many domains are unknown. Here we identify a conserved bacterial phosphoinositide-binding domain (BPD) that is found in functionally diverse Type III effectors of both plant and animal pathogens. We show that members of the BPD family functionally bind phosphoinositides and mediate localization to host membranes. Moreover, NMR studies reveal that the BPD of the newly identified Vibrio parahaemolyticus Type III effector VopR is unfolded in solution, but folds into a specific structure upon binding its ligand phosphatidylinositol-(4,5)-bisphosphate. Thus, our findings suggest a possible mechanism for promoting refolding of Type III effectors after delivery into host cells. Many Gram-negative bacterial pathogens manipulate host cellular processes to their advantage using effector proteins that are translocated into the host cell via the Type III Secretion System (T3SS) [1] , [2] . The T3SS is a syringe-like structure that delivers bacterial effectors across both bacterial and host membranes [3] . Translocation of effectors through the T3SS includes separation from the cognate bacterial chaperone, unfolding and ‘threading’ of the effectors through a needle complex [4] . Upon translocation into the host cell, effectors are thought to refold and carry out their function [4] . Notably, possible mechanisms that govern refolding inside the host cells remain unclear. Effectors must also find their cognate host target, and localization to a specific cell compartment helps to ensure their activity [5] . As many host targets of bacterial effectors are found on membranes, Type III effectors have evolved various strategies to target host membranes, such as host-mediated lipidation [5] and dedicated membrane-localization domains (MLD) [5] , [6] . However, the molecular mechanisms that mediate the membrane association of most of these MLDs have yet to be identified [5] , [6] . Vibrio parahaemolyticus is a Gram-negative marine bacterium that harbours two T3SSs (T3SS1 and T3SS2) [7] , and is a leading cause of gastroenteritis resulting from consumption of contaminated uncooked shellfish [8] . T3SS2 is found in clinical strains and is responsible for enterotoxicity and internalization into host cells [9] . T3SS1 is found in all tested strains and orchestrates a temporally regulated cell death [10] using three confirmed effectors: VopS, an AMPylator that inactivates Rho GTPases [11] ; VopQ, that forms a channel that disrupts host ion homoeostasis [12] ; and VPA0450, a phosphatidylinositol-5-phosphatase that depletes phosphatidylinositol-(4,5)-bisphosphate (PIP 2 ) from the plasma membrane (PM) and disrupts membrane integrity [13] . The T3SS1 gene cluster was previously suggested to encode additional effectors [14] , but these have yet to be experimentally confirmed. In this work, we find that one of the additional genes in the T3SS1 cluster, vp1683 , encodes a protein named VopR that is secreted via T3SS1 and localizes to the PM in eukaryotic cells. We identify an N-terminal domain required for this membrane localization and show that the molecular mechanism governing the PM localization is specific binding of a host phosphoinositide. Remarkably, the binding of this specific host ligand induces folding of the domain that is otherwise unfolded in solution, suggesting a mechanism that integrates both effector targeting and refolding after translocation into host cells. Complementation experiments reveal a similar phosphoinositide-binding domain in the V. parahaemolyticus effector VopS, and bioinformatic and functional analyses identify it as part of a family of bacterial phosphoinositide-binding domains (BPDs) found in diverse Type III effectors of both animal and plant pathogens. VopR localizes to PM via an N-terminal domain The gene vp1683 , found in the V. parahaemolyticus T3SS1 gene cluster, was previously suggested to encode a secreted Type III effector [14] , [15] . To determine whether vp1683 encodes a T3SS1 substrate, we monitored the secretion of a C-terminal FLAG-tagged VP1683. Indeed, we found that VP1683 (hereafter, VopR) was secreted from a strain harbouring a functional T3SS1 but not from a strain with a nonfunctional T3SS1 ( Supplementary Fig. S1a ). These results indicated that VopR is a secreted substrate of T3SS1. We next set out to determine the subcellular localization of VopR in eukaryotic cells. To do so, we monitored the localization of VopR fused to a C-terminal enhanced green fluorescent protein (eGFP) in yeast. We found that VopR specifically localized to the PM ( Fig. 1a ). Similar analyses of truncated VopR forms revealed that an N-terminal VopR 1–125 fragment was necessary and sufficient for the PM localization in yeast ( Fig. 1a and Supplementary Fig. S1b,c ). We next tested the localization of VopR in HeLa cells following transfection and found that, as in yeast, VopR localized to the PM via its N-terminal 125 amino acids ( Fig. 1b and Supplementary Fig. S1d ). 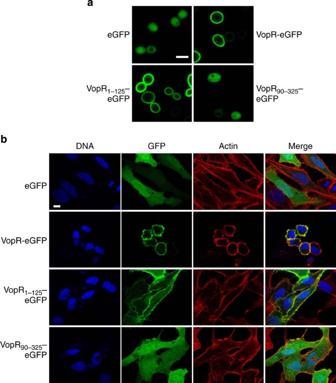Figure 1: VopR localizes to the PM. (a) Localization of galactose-inducible eGFP-fusion proteins in BY4741 yeast cells. Bar=5 μm. (b) Localization of eGFP-fusion proteins in transfected HeLa cells. Bar=10 μm. Figure 1: VopR localizes to the PM. ( a ) Localization of galactose-inducible eGFP-fusion proteins in BY4741 yeast cells. Bar=5 μm. ( b ) Localization of eGFP-fusion proteins in transfected HeLa cells. Bar=10 μm. Full size image Interestingly, expression of the full-length VopR resulted in HeLa cell rounding ( Fig. 1b ). To further characterize the effect of VopR on eukaryotic cells, we infected HeLa cells with V. parahaemolyticus strains deleted for all known T3SS1 effectors (i.e., VopQ, VopS, VPA0450 and VopR) or still expressing VopR. Infection with strains expressing VopR resulted in HeLa cell rounding, whereas this phenotype was not observed in the absence of VopR ( Supplementary Fig. S1e ). Thus, these results suggest that VopR is translocated into HeLa cells upon infection, where it both localizes to the membrane and induces cell rounding. VopR localizes to the PM via PIP 2 binding As several bacterial toxins have been shown to localize to host membranes via phospholipid-binding [5] , [6] , we next used a lipid overlay assay to test whether VopR bound phospholipids. We found that VopR specifically bound PIP 2 in vitro , and that VopR 1–125 was sufficient for this binding ( Fig. 2a ). To demonstrate the specificity of VopR for PIP 2 in vivo , we first tested the localization of VopR 1-125 in mss4 ts yeast at the non-permissive temperature (37 °C) in which PIP 2 is depleted from the PM [16] . We found that upon depletion of PIP 2 from the PM, VopR 1–125 was mostly cytoplasmic ( Fig. 2b ), as reported for the PIP 2 -binding PH domain of PLCδ (ref. 16 ). In addition, we expressed the eGFP-fused VopR 1–125 in HeLa cells followed by infection with a V. parahaemolyticus strain in which a T3SS2 regulator and all known T3SS1 effectors were deleted, except for the phosphatidylinositol-5-phosphatase VPA0450. Therefore, this strain only secretes the effector VPA0450, which was previously shown to deplete PIP 2 from the PM [13] . As shown in Fig. 2c , removal of PIP 2 from the PM by VPA0450 resulted in the loss of VopR 1–125 PM localization. We thus concluded that the molecular mechanism governing VopR localization to the PM is specific binding of PIP 2 by an N-terminal domain, which we named BPD. 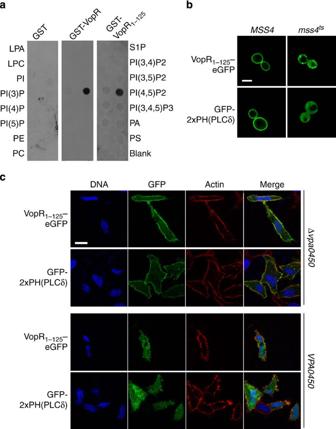Figure 2: VopR1–125specifically binds PIP2. (a) Lipid overlay assay with purified GST-fusion proteins. Membranes were immunoblotted with anti-GST antibodies. (b) Localization of galactose-inducible proteins inMSS4wild-type or temperature-sensitive mutant yeast at the restrictive temperature (37 °C). Bar=5 μm. (c) Localization of indicated proteins in transfected HeLa cells 2 h post infection withVibriostrains expressing (bottom panels), or deleted for (top panels),vpa0450. Bar=10 μm. Figure 2: VopR 1–125 specifically binds PIP 2 . ( a ) Lipid overlay assay with purified GST-fusion proteins. Membranes were immunoblotted with anti-GST antibodies. ( b ) Localization of galactose-inducible proteins in MSS4 wild-type or temperature-sensitive mutant yeast at the restrictive temperature (37 °C). Bar=5 μm. ( c ) Localization of indicated proteins in transfected HeLa cells 2 h post infection with Vibrio strains expressing (bottom panels), or deleted for (top panels), vpa0450 . Bar=10 μm. Full size image PIP 2 -binding induces specific folding for BPD VopR To further characterize the BPD VopR , we purified VopR 1–125 fused to N-terminal His 6 and Gβ1 tags for improved solubility and purification. This protein eluted as a single peak from size exclusion chromatography, which inline multi-angle laser light scattering (SEC-MALLS, size exclusion chromatography-multi-angle laser light scattering) confirmed as having the molecular weight of a monomeric fusion protein (23 kDa; Supplementary Fig. S2a ). To gain some insight into BPD VopR structure and interactions, we used solution NMR to examine the effects of ligand binding on purified His-Gβ1-VopR 1–125 . Alone, the spectrum of His-Gβ1-VopR 1–125 chiefly contained peaks that could be attributed to the N-terminal Gβ1 domain; most of the remaining peaks originating from VopR 1–125 had heterogenous line widths and poor 1 H chemical shift dispersion, consistent with unfolding ( Fig. 3a ). Moreover, the protein precipitated rapidly at 25 °C ( Supplementary Fig. S2b ). Remarkably, addition of PIP 2 to His-Gβ1-VopR 1–125 , but not other phosphoinositides, substantially improved both NMR spectra (including the appearance of many new well-resolved peaks) ( Fig. 3b and Supplementary Fig. S2c–f ) and solubility ( Supplementary Fig. S2b ). These results indicated that the BPD VopR is unstructured in solution without a phosphoinositide ligand, but that specific binding of PIP 2 induces its folding. Further analysis using circular dichroism (CD) spectroscopy revealed a PIP 2 -dependent increase in secondary structure within His-Gβ1-VopR 1–125 , corroborating these findings ( Supplementary Fig. S3 ). 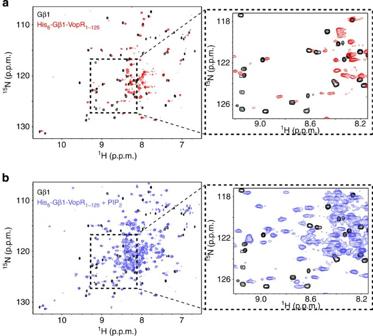Figure 3: PIP2induces VopR1–125folding in solution. (a)15N/1H HSQC spectra of Gβ1 (black) and His6-Gβ1-VopR1–125(red). (b)15N/1H HSQC spectra of Gβ1 (black) and His6-Gβ1-VopR1–125(blue) in the presence of PI(4,5)P2-diC8 (at 1:1 molar ratio). Dashed line indicates region shown in expansion on right. All spectra were recorded at 25 °C on a 600 MHz NMR with VopR samples at 200 μM protein. Figure 3: PIP 2 induces VopR 1–125 folding in solution. ( a ) 15 N/ 1 H HSQC spectra of Gβ1 (black) and His 6 -Gβ1-VopR 1–125 (red). ( b ) 15 N/ 1 H HSQC spectra of Gβ1 (black) and His 6 -Gβ1-VopR 1–125 (blue) in the presence of PI(4,5)P 2 -diC8 (at 1:1 molar ratio). Dashed line indicates region shown in expansion on right. All spectra were recorded at 25 °C on a 600 MHz NMR with VopR samples at 200 μM protein. Full size image The N-terminus of VopS functionally complements BPD VopR Having established that the BPD VopR is responsible for PM localization via PIP 2 binding, we asked whether it is required for VopR-mediated cell rounding. To test this, we employed an effector-less Yersinia strain as a heterologous system that translocates Vibrio Type III effectors [17] and monitored the rounding of HeLa cells by a truncated VopR 90–325 protein that does not contain an intact BPD. Since the Yersinia T3SS can only secrete effectors that contain the N-terminal secretion signal (missing in the VopR 90–325 truncation), we swapped the N-terminal 90 amino acids of VopR with those of two other Vibrio effectors (VopQ and VopS) to allow VopR 90–325 secretion ( Supplementary Fig. S4a ). Infection with a Yersinia strain expressing the VopQ 1–90 –VopR 90–325 fusion did not cause cell rounding, indicating that the BPD is required for this VopR-mediated phenotype ( Fig. 4a ). Surprisingly, infection with the VopS 1–90 –VopR 90–325 expressing strain resulted in cell rounding ( Fig. 4a ). The ability of the VopS N-terminus to complement the VopR BPD truncation in this assay prompted us to examine whether the N-terminus of VopS also complemented the BPD-mediated PM localization of VopR. Indeed, the VopS 1–90 –VopR 90–325 fusion localized to the PM ( Fig. 4b and Supplementary Fig. S4b,c ), while the VopQ 1–90 –VopR 90–325 fusion did not ( Supplementary Fig. S4b,c ). These results led us to hypothesize that the N-terminus of VopS encodes a PM-targeting signal. In agreement with this proposal, we found that VopS localized to the PM in yeast ( Fig. 4c ) and HeLa cells ( Supplementary Fig. S8c ), as did VopS 1–125 ( Fig. 4c,d and Supplementary Fig. S4d,e ). 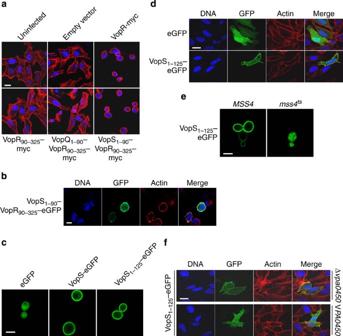Figure 4: VopS contains a PIP2-binding BPD. (a) HeLa cells 5 h after infection with effector-lessYersiniainduced to express the indicated proteins. Actin (red) and DNA (Blue) are shown. Bar=20 μm. (b) Localization of eGFP-fusion protein in transfected HeLa cells. Bar=10 μm. (c) Localization of galactose-inducible eGFP-fusion proteins in BY4741 yeast cells. Bar=5 μm. (d) Localization of eGFP-fusion proteins in transfected HeLa cells. Bar=10 μm. (e) Localization of galactose-inducible VopS1–125–eGFP inMSS4wild-type or temperature-sensitive mutant yeast at the restrictive temperature (37 °C). Bar=5 μm. (f) Localization of VopS1–125–eGFP in transfected HeLa cells 2 h after infection withVibriostrains expressing (bottom panel), or deleted for (top panel),vpa0450. Bar=10 μm. Figure 4: VopS contains a PIP 2 -binding BPD. ( a ) HeLa cells 5 h after infection with effector-less Yersinia induced to express the indicated proteins. Actin (red) and DNA (Blue) are shown. Bar=20 μm. ( b ) Localization of eGFP-fusion protein in transfected HeLa cells. Bar=10 μm. ( c ) Localization of galactose-inducible eGFP-fusion proteins in BY4741 yeast cells. Bar=5 μm. ( d ) Localization of eGFP-fusion proteins in transfected HeLa cells. Bar=10 μm. ( e ) Localization of galactose-inducible VopS 1–125 –eGFP in MSS4 wild-type or temperature-sensitive mutant yeast at the restrictive temperature (37 °C). Bar=5 μm. ( f ) Localization of VopS 1–125 –eGFP in transfected HeLa cells 2 h after infection with Vibrio strains expressing (bottom panel), or deleted for (top panel), vpa0450 . Bar=10 μm. Full size image Notably, while the amino-acid sequences of the VopR and VopS N-termini had limited similarity, we found that they share similar predicted secondary structures ( Fig. 5a and Supplementary Fig. S5 ). Therefore, we speculated that the N-terminus of VopS also contains a PIP 2 -binding BPD. To test this, we monitored the localization of a VopS 1–125 –eGFP fusion in mss4 ts mutant yeast. We found that similar to BPD VopR , VopS 1–125 lost its PM localization in mss4 ts mutant yeast at the non-permissive temperature ( Fig. 4e ). Moreover, expression of a VopS 1–125 –eGFP fusion in HeLa cells in the presence of the phosphatidylinositol-5-phosphatase VPA0450 also resulted in loss of the PM localization ( Fig. 4f ). Taken together, these results suggest that VopR and VopS both contain functional N-terminal PIP 2 -binding BPDs. 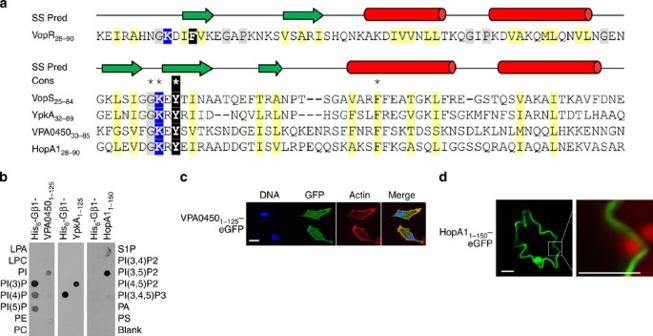Figure 5: BPDs of VPA0450, YpkA, and HopA1 bind phosphoinositides and localize to eukaryotic membranes. (a) The ‘core’ region of the VopR (GI:28898457) BPD (top), and the VopS (GI:28898460), VPA0450 (GI:28900305), YpkA (GI:51593847) and HopA1 (GI:28872465) aligned BPDs (bottom), with corresponding secondary structure prediction shown above: α-helices (red) and β-strands (green); and functional sequence motif indicated by asterisks. Conserved residues are highlighted yellow (mainly hydrophobic), grey (small), polar motif (blue) and functional motif (black). (b) Lipid overlay assay with purified His6-Gβ1-fusion proteins. Membranes were immunoblotted with anti-His antibodies. (c) Localization of eGFP-fusion protein in transfected HeLa cells. Bar=10 μm. (d) Localization of eGFP-fusion protein inAgrobacterium-infiltrated tomato epidermal cells. White box indicates region shown in expansion on the right. Chloroplast auto-fluorescence (red) is shown in right panel. Bar=10 μm. Figure 5: BPDs of VPA0450, YpkA, and HopA1 bind phosphoinositides and localize to eukaryotic membranes. ( a ) The ‘core’ region of the VopR (GI:28898457) BPD (top), and the VopS (GI:28898460), VPA0450 (GI:28900305), YpkA (GI:51593847) and HopA1 (GI:28872465) aligned BPDs (bottom), with corresponding secondary structure prediction shown above: α-helices (red) and β-strands (green); and functional sequence motif indicated by asterisks. Conserved residues are highlighted yellow (mainly hydrophobic), grey (small), polar motif (blue) and functional motif (black). ( b ) Lipid overlay assay with purified His 6 -Gβ1-fusion proteins. Membranes were immunoblotted with anti-His antibodies. ( c ) Localization of eGFP-fusion protein in transfected HeLa cells. Bar=10 μm. ( d ) Localization of eGFP-fusion protein in Agrobacterium -infiltrated tomato epidermal cells. White box indicates region shown in expansion on the right. Chloroplast auto-fluorescence (red) is shown in right panel. Bar=10 μm. Full size image A BPD family identified in Type III effectors We next set out to identify additional BPD-containing Type III effectors using iterative BLAST methods. Using the BPD of VopS as a template for these searches, we identified three additional confirmed effectors with predicted BPDs at their N-termini: the V. parahaemolyticus VPA0450 (ref. 13 ); the Yersinia YpkA (also referred to as YopO) [18] ; and the phytopathogen Pseudomonas syringae HopA1 (ref. 19 ) ( Fig. 5a and Supplementary Fig. S5b ). Interestingly, the BPDs of these three effectors, BPD VopS and BPD VopR all share a similar predicted secondary structure consisting of two β-strands followed by two α-helices that align to form the BPD ‘core’ ( Fig. 5a and Supplementary Fig. S5 ). This secondary structure prediction was supported by NMR analysis of PIP 2 -bound VopR 1–125 that confirmed the presence of both predicted β-strands (VopR residues 37–42 and 47–56) and both predicted α-helices (VopR residues 60–69 and 78–84) in the folded state ( Supplementary Fig. S6 ). BPD VopS , BPD VPA0450 , BPD YpkA and BPD HopA1 also share a conserved GKxY motif in their second β-strand and an invariant F in the first α-helix ( Fig. 5a and Supplementary Fig. S5b ). To verify that BPD VPA0450 , BPD YpkA and BPD HopA1 are functional, we tested their ability to bind phosphoinositides using a lipid overlay assay. We found that all three bound phosphoinositides in vitro ( Fig. 5b ). We next determined the subcellular localizations of these BPDs. BPD VPA0450 partially localized to the PM in HeLa cells ( Fig. 5c ) and to the PM and an internal membrane in yeast ( Supplementary Fig. S7a,c ). BPD YpkA overlaps with the previously described MLD of YpkA that localizes to the PM in mammalian cells [20] , as we similarly found in yeast ( Supplementary Fig. S7b,c ). In HopA1, we identified amino acids 1–150 (BPD HopA1 ) as a region functionally equivalent to the other BPDs that partially localized to the yeast PM ( Supplementary Fig. S7d,e ), and to the PM and nucleus in tomato epidermal cells ( Fig. 5d ). Taken together, these results support the proposal that the BPD is a phosphoinositide binding domain that is common to Type III effectors of both animal and plant pathogens. Conserved motif required for membrane localization of BPDs To gain further insight into the mechanism of phosphoinositide-binding by BPDs, we mutated several residues of the conserved GKxYx n F motif shared among BPD VopS , BPD VPA0450 , BPD YpkA and BPD HopA1 ( Fig. 5a ) and tested their effects on the PM localization. Within VopS, we found that a mutation in Tyr34, central to this motif and predicted to be in the first β-strand of the BPD VopS ‘core’, abolished the PM localization in yeast and in HeLa cells ( Fig. 6a and Supplementary Fig. S8c ) but did not hamper the toxicity of VopS ( Supplementary Fig. S8 ). The catalytically inactive mutant VopS H348A , which is unable to AMPylate substrates [11] , was used as a negative control in these experiments. Mutations in the conserved tyrosines of BPD VPA0450 and BPD HopA1 also resulted in loss of membrane localization in yeast ( Fig. 6b ), confirming a functional role for the sequence motif. Unfortunately, we were unable to detect expression of a Tyr41-mutated form of BPD YpkA , suggesting that it may play an integral role in the proper folding of this domain. Notably, an isoleucine (Ile38) is found in VopR in place of the tyrosine that is conserved in the other family members ( Fig. 5a ). Mutation in this isoleucine resulted in partial mislocalization of BPD VopR to the cytoplasm in yeast ( Fig. 6b ). 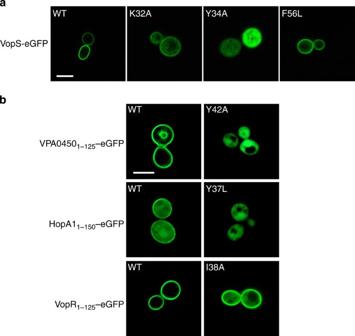Figure 6: A conserved motif required for membrane localization of BPDs. Localization of galactose-inducible eGFP-fusion proteins in BY4741 yeast cells. WT, wild-type protein. Bar=5 μm. (a) Localization of VopS mutations. (b) Localization of BPDVPA0450, BPDHopA1and BPDVopRmutants. Figure 6: A conserved motif required for membrane localization of BPDs. Localization of galactose-inducible eGFP-fusion proteins in BY4741 yeast cells. WT, wild-type protein. Bar=5 μm. ( a ) Localization of VopS mutations. ( b ) Localization of BPD VPA0450 , BPD HopA1 and BPD VopR mutants. Full size image Phosphoinsitide-binding domains often use cationic residues to bind the negatively charged phosphates [6] . Because the only cationic residue that is conserved in all BPDs was not required for membrane localization of VopS (Lys32, Fig. 6a ), we tested the effect of mutations in less conserved cationic residues on the membrane localization of BPD VopS in yeast. We found that three partially conserved residues (Arg45, Lys62 and Arg65) were required for PM localization ( Supplementary Fig. S9 ). Bacterial toxins that function inside the host cell, such as Type III effectors, need to localize to the correct intracellular compartment or membrane to carry out their functions. Here we identified the first family of BPD that is shared by diverse Type III effectors of both animal and plant pathogens. Furthermore, we presented evidence supporting a possible mechanism for refolding of Type III effectors upon translocation into the host cell, coupled with targeting to the appropriate cellular compartment. In addition to the previously identified T3SS1 effectors of V. parahaemolyticus (VopS, VopQ and VPA0450), we found that VopR is also secreted via T3SS1. The heterologous Yersinia pseudotuberculosis T3SS was able to secrete VopR, dependent on an intact N-terminus that contains the putative Type III secretion signal. We also showed that transient expression of VopR in HeLa cells resulted in cell rounding, and that a similar cell rounding phenotype was observed when HeLa cells were infected with V. parahaemolyticus expressing VopR. Thus, we conclude that VopR was not only secreted but actually translocated into the eukaryotic cell by the T3SS, where it induced cell rounding. Using several different methods, we showed that the N-terminus of VopR (BPD VopR ) specifically binds PIP 2 to localize to the eukaryotic PM. Remarkably, it appears that the BPD VopR is unfolded and quickly precipitates in solution, but folds into a specific soluble structure upon binding PIP 2 . Interestingly, Letzelter et al . [20] previously suggested that the N-terminal chaperone-binding domains and MLDs of Type III effectors overlap to allow the chaperones to mask aggregation-prone host-localization domains inside the bacterium. While Type III effectors need to be unfolded during translocation through the T3SS, they are folded inside the bacterium and in the host cell [21] . Our findings suggest a possible mechanism for Type III effectors refolding after delivery. We propose a model in which chaperones bind to otherwise unstructured host-localization domains of Type III effectors while inside the bacterium. The effectors are then separated from the chaperones and unfold to allow translocation through the T3SS. Once inside the eukaryotic host cell, the unfolded effectors can recognize a specific ligand found in the eukaryotic host cell, and this binding induces their refolding ( Fig. 7 ). In VopR, the ligand PIP 2 also serves as a mechanism for subcellular localization. Unfortunately, low expression levels, solubility and stability of other BPDs prevented the expansion of this model to additional BPD-containing effectors. Notably, a ligand-induced folding was previously reported for the epsin ENTH domain in which a new helix became ordered upon binding of inositol-1,4,5-trisphosphate [22] . 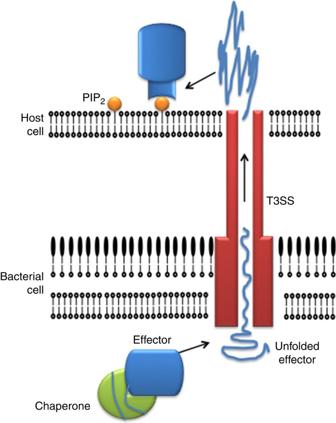Figure 7: Model for Type III effectors refolding and targeting in host cells. Chaperones (Green ball) bind to otherwise unstructured host-localization domains of Type III effectors (Blue strand) to prevent aggregation while inside the bacterium. To translocate through the T3SS (Red cylinders), effectors are separated from the chaperones and must unfold to allow passage through the ‘needle’ structure. Once inside the host cell, the unfolded effectors can bind a host-specific ligand (Yellow ball; in this case PIP2on the PM) and promote both refolding of the effector (Blue cylinder) and localization to the appropriate cellular compartment. Figure 7: Model for Type III effectors refolding and targeting in host cells. Chaperones (Green ball) bind to otherwise unstructured host-localization domains of Type III effectors (Blue strand) to prevent aggregation while inside the bacterium. To translocate through the T3SS (Red cylinders), effectors are separated from the chaperones and must unfold to allow passage through the ‘needle’ structure. Once inside the host cell, the unfolded effectors can bind a host-specific ligand (Yellow ball; in this case PIP 2 on the PM) and promote both refolding of the effector (Blue cylinder) and localization to the appropriate cellular compartment. Full size image The ability of the VopS N-terminus to complement the VopR-mediated rounding phenotype in HeLa cells as well as the PM localization of the VopR 90–325 truncation prompted us to hypothesize and subsequently show that VopS also contains a functional PIP 2 -binding BPD. Using bioinformatic and functional analyses, these findings led us to identify the Type III effectors VPA0450, YpkA and HopA1 as additional members of a broader BPD family. While isolated examples of Type III effectors that contain a phosphoinositide binding domain have been previously reported (e.g., the Pseudomonas aeruginosa Type III effector ExoU [5] , [23] ), this is, to the best of our knowledge, the first report of a phosphoinositide binding domain family that is shared between functionally diverse effectors of both plant and animal bacterial pathogens. Moreover, this is the first report of a phytopathogen Type III effector (i.e., HopA1) that binds phosphoinositides. Interestingly, PIP 2 appears to be a ‘hub’ for V. parahaemolyticus T3SS1 effectors, as both VopR and VopS use it to localize to the PM, and it is hydrolysed and depleted from the PM by VPA0450 (ref. 13 ). It is therefore possible that VPA0450 serves as a temporal regulator of VopR and VopS activities on the host PM. For the Yersinia effector YpkA, the N-terminus was previously reported to be an MLD (overlapping with the BPD described in this work). However, the mechanism governing its PM localization was unknown [20] . Our result revealed that this MLD is in fact a member of the BPD family that localize to host membranes via phosphoinositide binding. It should be noted that, although all the BPDs appeared to functionally bind phosphoinositides in vitro , a more detailed analysis will be required to determine their actual physiological-binding specificities. While the BPDs share limited amino-acid sequence similarity, our analysis of the secondary structure predictions for the BPDs revealed a common ‘core’ that consists of two β-strands followed by two α-helices. Similar characteristics can be found in eukaryotic phosphoinositides binding domain, as Phox domains show weak primary sequence identity but have a conserved secondary structure of three β-strands followed by three α-helices [24] . Using NMR analysis, we confirmed the prediction for the PIP 2 -bound BPD VopR secondary structure. Moreover, we showed that a tyrosine residue conserved in the BPDs of VopS, VPA0450, YpkA and HopA1 is required for membrane localization. While this residue may be part of the phosphoinositide binding pocket, its position in the middle of a β-strand could suggest that it has a role in maintaining the BPD structure. In addition, we identified three cationic residues in the BPD VopS that were required for PM localization in yeast, suggesting that they may participate directly in phosphoinositide binding. Notably, the BPD HopA1 ‘core’ corresponds exactly with its secretion-translocation signal, for which a structure bound to its bacterial chaperone was recently published [25] . Importantly, the BPD HopA1 wraps around the chaperone, assuming a non-globular structure from secondary structure elements that are consistent with our prediction [25] . While the BPDs share common themes with other bacterial MLDs, such as being rich in Leu/Ile residues, containing multiple charged residues and having at least one conserved hydrophobic residue [6] , the BPD secondary structure is unique and thus defines a distinct new domain. Moreover, the secondary structure of the BPD is also distinct from those of known eukaryotic BPDs [26] , suggesting that the BPD is the result of convergent evolution. The localization to the PM via PIP 2 binding was required for the VopR-mediated rounding of HeLa cells. Similarly, the BPD YpkA (MLD) was previously shown to be required for YpkA-mediated cell rounding and PM localization [20] . Therefore, the BPD-mediated PM localization is required for VopR and YpkA toxic effects inside the host cell. Surprisingly, however, VopS did not require its BPD-mediated PM localization to induce its toxic effects in eukaryotic cells, suggesting that the requirement for BPD-mediated membrane localization is not shared by all BPD-containing Type III effectors. In summary, we identified a new family of Type III effectors, from both animal and plant pathogens, containing a BPD that mediates membrane localization. These studies exemplify the compact and malleable nature of bacterial T3SS effectors that are secreted to efficiently target their host substrates. Strains and media Escherichia coli strain DH5α was used for routine cloning and plasmid amplification and was grown in Luria-Bertani (LB) broth or 2xYT broth at 37 °C. The V. parahaemolyticus RIMD 2210633 derivative strain POR1 (RIMD 2210633 Δ tdhAS) [27] was used to construct strains POR1 (Δ vtrA , Δ vopS , Δ vopQ and Δ vpa0450 ), POR1 (Δ vtrA , Δ vopS , Δ vopQ and Δ vopR ) and POR1 (Δ vtrA , Δ vopR , Δ vopQ and Δ vpa0450 ), referred to as VopR , VPA0450 and VopS , respectively. POR1 (Δ vtrA , Δ vopS , Δ vopQ , Δ vopR and Δ vpa0450 ) is used as a control strain lacking all four known T3SS1 effectors and is referred to as Δ vopR , Δ vpa0450 or Δ vopS , where appropriate. Strain POR2 (POR1 Δ vcrD1 ) was used as a T3SS1-deficient strain (T3SS1−) [27] . Vibrio strains were grown in LB medium supplemented with 2% NaCl (MLB) at 30 °C (ref. 28 ). The effector-less Y. pseudotubrculosis strain YP37 [29] was grown in 2xYT broth at 23 °C. Agrobacterium tumefaciens strain GV2260 was grown in 2xYT broth at 30 °C. Yeast strains used were BY4741 (MATa his3Δ0 leu2Δ0 met15Δ0 ura3Δ0), and the strains SEY6210 ( MAT α leu2-3,112 ura3-52 his3- Δ 200 trp1- Δ 901 suc2- Δ 9 lys2-801; GAL ) and AAY202 (SEY6210: mss4 ts ) referred to as MSS4 and mss4 ts , respectively [16] . HeLa cells (ATCC) were maintained in DMEM (Invitrogen) supplemented with 10% heat-inactivated fetal bovine serum (Sigma), sodium pyruvate, penicillin/streptomycin/glutamine (Invitrogen) and 5% CO 2 . Plasmids For yeast expression and localizations, the e GFP gene was cloned into the EcoRI site in pGMU10 (RIKEN) in-frame with the C-terminal myc tag to produce pDGFP. The vopR , vopS and vpa0450 genes from V. parahaemolyticus RIMD 2210633 were PCR cloned in-frame with the eGFP–myc into pDGFP XbaI and SacI sites. The hopA1 gene from P. syringae DC3000 and the ypkA gene from Y. pseudotuberculosis were PCR cloned in-frame with the eGFP–myc into pDGFP XbaI and KpnI sites. For HeLa cells expression and localizations, eGFP–myc fusions from pDGFP were PCR amplified and cloned into HindIII and NotI sites in pSFFV (Addgene). For expression and localizations in tomato, the hopA1 gene was cloned from pGML10:HopA1 (ref. 30 ) into the XbaI and BamHI sites in the binary vector pBINPLUS in-frame with the e GFP gene [31] . For secretion from V. parahaemolyticus , the vopR gene from V. parahaemolyticus RIMD 2210633 was PCR cloned in-frame with a C-terminal FLAG tag into the SacI site in pBAD/ Myc-His (Invitrogen) and downstream to the 1,000 bp that are found of the V. parahaemolyticus RIMD 2210633 vp1393 for constitutive expression. For VopS secretion, the vopS gene including the 1,000 bp upstream of the ATG start codon from V. parahaemolyticus RIMD 2210633 was PCR amplified and cloned into NcoI and HindIII sites in pBAD2 (ref. 32 ) with a stop codon to avoid the C-terminal tag. For infections with V. parahaemolyticus , the vopR gene including the 667 bp upstream of the ATG start codon from V. parahaemolyticus RIMD 2210633 was PCR cloned into XhoI and HindIII sites in pBAD/ Myc-His . For expression and secretion from Y. pseudotuberculosis , the vopR gene or a truncated version encoding amino acids 90–325 from V. parahaemolyticus RIMD 2210633 were PCR cloned in-frame with a C-terminal myc tag into XbaI and KpnI sites in pMMB67HE (Addgene). To generate the effectors-fusion constructs, the vopS and vopQ genes encoding amino acids 1–90 from V. parahaemolyticus RIMD 2210633 were PCR cloned upstream of the truncated vopR into HindIII and XbaI sites. For protein expression and purification, the vopR gene or a truncated version encoding amino acids 1–125 from V. parahaemolyticus RIMD 2210633 were PCR cloned downstream of glutathione S -transferase (GST) into BamHI and XhoI sites in the pGex-rTEV (NEB). Truncated versions of vpa0450 , ypkA and hopA1 were PCR cloned downstream of His 6 -Gβ1 into EcoRI and NotI sites in the pHis-Gβ1 Parallel vector [33] , whereas vopR truncation was clones into EcoRI and XhoI sites. Primers used for cloning are listed in Supplementary Table S1 . Site-specific mutations were introduced using the QuikChange kit (Stratagene) following the manufacturer’s instructions. Primers used for mutagenesis are listed in Supplementary Table S2 . Construction of deletion strains In-frame deletions were performed by cloning the nucleotide sequences 1 kb upstream and 1 kb downstream of vtrA ( vpa1332 ), vopR ( vp1683 ), vopS ( vp1686) , vopQ ( vp1680 ) and vpa0450 into pDM4, a Cm R OriR6K suicide plasmid. The resulting plasmids were conjugated into the POR1 strain or its derivatives from E . coli S17 (λ pir) and transconjugants were selected on media containing 25 μg ml −1 chloramphenicol. Bacteria were counter-selected by growing on media containing 15% sucrose. Deletions and insertions were confirmed by PCR. Yeast transformation and induction Yeast transformations were performed using the LiAc method [34] . For galactose-inducible expression, cells were grown overnight at 30 °C in glucose-containing (2%) media. Cells were washed twice with water and diluted 10-fold in galactose and raffinose containing media (2% and 1%, respectively) and grown at 30 °C for 8–12 h. For depletion of PIP 2 from the PM in the mss4 ts strain, cells were incubated at the restrictive temperature (37 °C) for 45 min. Transfections and infections For transfection of HeLa cells, 1 × 10 5 cells were seeded on sterile coverslips in six-well dishes and grown for 24 h. Cells were transfected with FuGENE HD (Roche) transfection reagent using 0.2 μg of the appropriate plasmid. Empty pSFFV vector was added for a total of 2 μg DNA per well. Eighteen to twenty hours after transfection, cells were fixed and stained as indicated. For Vibrio infections, Vibrio strains were incubated in DMEM for 30 min at 37 °C before infection, to induce type III secretion. Multiplicity of infection=10 [13] . Before infection (multiplicity of infection=10), Yersinia strains were incubated in LB containing 20 mM sodium oxalate and 10 mM magnesium chloride for 1 h at 23 °C to induce type III secretion, followed by addition of 400 μM isopropyl-β- D -thiogalactoside (IPTG) and transfer to 37 °C for 1.5 h. For Agrobacterium infiltrations into tomato leaves for transient protein expression Agrobacterium cultures were grown overnight at 30 °C in LB broth with the appropriate antibiotics and washed in infiltration medium (10 mM morpholinoethanesulfonic acid, 10 mM MgCl 2 and 0.2 mM acetosyringone). Agrobacterium cultures were normalized to a final OD 600 =0.06 and infiltrated into leaves [35] . Secretion assays V. parahaemolyticus strains were grown in MLB overnight at 30 °C, washed and diluted 1:10 into prewarmed DMEM and incubated for 3 h at 37 °C. Y. pseudotuberculosis strains were grown in 2xYT overnight, diluted 1:10 into LB containing 20 mM sodium oxalate and 10 mM magnesium chloride and grown for 1 h at 23 °C to induce type III secretion. IPTG (400 μM) was added and cells were shifted to 37 °C for 4 h. One OD 600 units were collected for cell protein analysis. The supernatant of 10 OD 600 units was collected for medium protein analysis. Supernatants were filtered and precipitated with deoxycholate (150 μg ml −1 ) and trichloroacetic acid (6% v/v). Precipitated proteins were pelleted and washed with acetone, before resuspension in 40 μl of 2x Laemmli sample buffer [32] . Confocal microscopy HeLa cells were fixed in 3.2% paraformaldehyde after treatment. Nuclei were stained with Hoechst (Sigma), and the actin cytoskeleton was stained with Rhodamine-phalloidin or Alexa488-phalloidin (Molecular Probes). Yeast cultures were washed and resuspended in 10 mM Tris (pH 8.0) before mounted on slides. MSS4 and mss4 ts were pretreated at 37 °C for 45 min. Tomato leaf slices (5 × 5 mm) were placed in water on slides. Samples were viewed on a Zeiss LSM 510 scanning confocal microscope. Lipid overlay assays Pre-spotted PIP strips (Echelon Biosciences) were used following the manufacturer’s instructions. GST fusion proteins were detected using anti-GST antibodies (1:1,000 dilution) (Covance). His 6 -Gβ1-fusion proteins were detected using anti-His antibodies (1:1,000 dilution) (Invitrogen). Cell lysis and immunoblotting For yeast cell lysis, 1 ml of galactose-induced cultures were collected, cells were harvested and resuspended in 100 μl ice-cold lysis solution (4% v/v 5 N NaOH, 0.5% v/v β-mercaptoethanol) and incubated on ice for 30 min. Lysates were titrated to pH of 9–10 using HCl and 2x Laemmli sample buffer was added. HeLa cells were collected from a transfected six-well, washed twice with phosphate-buffered saline (pH 7.5) and boiled in 2x Laemmli sample buffer. Proteins were resolved on SDS–polyacrylamide gel electrophoresis and transferred to polyvinylidene difluoride membranes. Protein expression in yeast was detected using anti-myc antibodies (1:1,000 dilution) (9E10, SC-40) (Santa Cruz) [34] . Protein expression in HeLa cells was detected using anti-GFP antibodies (1:1,000 dilution) (Clontech) or anti-VopS antibodies (1:1,000 dilution) [11] . Bioinformatics PSI-BLAST [36] searches were initiated using the VopS N-terminus (GI|28898460:1–100) as a query against the NR database, with default parameters and E -value cutoff 0.01. The N-terminus of YpkA (GI|145301479) was detected in the second iteration with E -value 0.004, and the N-terminus of HopA1 was detected in the third iteration with a marginal E -value. Transitive PSI-BLAST searches were performed with all identified N-terminal effector sequences as queries. HopA1 queries identified VPA0450 and VopS N-termini. Multiple sequence alignments were done using PROMALS [37] , with manual adjustments based on PSI-BLAST [36] alignments, secondary structure predictions from the JPRED3 server [38] , and positional conservations viewed using Jalview [39] . Protein purification and size exclusion chromatography pGex-rTEV and pHis-Gβ1 vectors were transformed into BL21 (DE3) (Novagen), grown in 2xYT and induced with 400 μM IPTG. His-tagged proteins (His 6 -Gβ1-VopR 1–125 , His 6 -Gβ1-VPA0450 1–125 , His 6 -Gβ1-YkpA 1–125 and His 6 -Gβ1-HopA1 1–150 ) were purified with the use of Ni 2+ affinity purification (Qiagen). GST-tagged proteins (GST-VopR and GST-VopR 1–125 ) were purified with the use of glutathione agarose beads (Sigma). For NMR analysis, purified His 6 -Gβ1-VopR 1–125 was loaded onto a Superdex 75 16/60 (GE Healthcare) equilibrated with 25 mM Tris (pH 7.5), 100 mM NaCl and elution was monitored via absorbance at 280 nm. The molecular mass of apo state His 6 -Gβ1-VopR 1–125 was determined with SEC-MALLS by injecting 500 μl of 60 μM protein onto a Superdex 75 10/300 analytical gel filtration column connected with a mini-DAWN Treos static light scattering instrument (Wyatt) and an in-line refractive index detector. Molar mass was calculated using Wyatt Astra software. Solution NMR spectroscopy For NMR studies, isotopically labelled samples of His 6 -Gβ1-VopR 1-125 were produced from BL21 (DE3) cultures grown in M9 media supplemented with 1 g l −1 15 NH 4 Cl and 3 g l −1 U- 13 C 6 -glucose (Cambridge Isotope Labs) as the sole nitrogen and carbon sources as needed. Proteins were expressed overnight at 23 °C and purified with the use of Ni 2+ affinity (Qiagen) and Superdex 75 gel filtration (GE Healthcare) chromatography, as described above, for additional purification. Proteins were concentrated to 200–400 μM in 25 mM Tris (pH 7.5), 100 mM NaCl buffer. All NMR experiments were carried out at 25 °C on cryoprobe-equipped Varian Inova 600 MHz spectrometers. Ligand binding was monitored with 15 N/ 1 H HSQC (Heteronuclear Single-Quantum Correlation) experiments on uniformly 15 N labelled protein samples [40] . When indicated, the phosphoinositides PI(4,5)P 2 -diC8, PI(3)P-diC8 or PI(3,4,5)P 3 -diC8 (Echelon Biosciences) were added at a 1:1 molar ratio to the protein. Backbone chemical shift assignments used standard methods (HNCACB, CBCA(CO)NH, HNCO and (H)C(CO)NH-TOCSY) [40] on a 350 μM sample of uniformly 15 N/ 13 C His 6 -Gβ1-VopR 1-125 in buffer containing PI(4,5)P 2 -diC8 at a 1:1 molar ratio (from a 5 mM stock solution) (Echelon Biosciences), 25 mM Tris (pH 7.5), 100 mM NaCl, 10% D 2 O supplemented with 6 μg His 6 -TEV protease to free VopR from the His 6 -Gβ1 fusion partner in situ . All NMR data were processed with NMRpipe/NMRDraw [41] and analysed with NMRviewJ (One Moon Scientific), allowing us to establish backbone chemical shift assignments for 34% of residues in the BPD. Secondary structure analyses were generated by TALOS-N [42] from our backbone chemical shift assignments. CD spectroscopy CD spectra were collected on a J-815 CD spectrometer using a 0.1 cm path length cuvette, using 10 μM His 6 -Gβ1-VopR 1-125 protein titrated with various concentrations of PI(4,5)P 2 -diC8 in 25 mM Tris (pH 7.5), 100 mM NaCl at 4 °C. Spectra were recorded every 0.1 nm from 200 to 250 nm with triplicate scans. Molar residue ellipticities (deg-cm 2 per dmol-res) were calculated from raw ellipticities (mdeg). How to cite this article: Salomon, D. et al . Effectors of animal and plant pathogens use a common domain to bind host phosphoinositides. Nat. Commun. 4:2973 doi: 10.1038/ncomms3973 (2013).